Relation between the nodal and antinodal gap and critical temperature in superconducting Bi2212 An energy gap is, in principle, a dominant parameter in superconductivity. However, this view has been challenged for the case of high- T c cuprates, because anisotropic evolution of a d -wave-like superconducting gap with underdoping has been difficult to formulate along with a critical temperature T c . Here we show that a nodal-gap energy 2Δ N closely follows 8.5 k B T c with underdoping and is also proportional to the product of an antinodal gap energy Δ * and a square-root superfluid density √ P s for Bi 2 Sr 2 CaCu 2 O 8+ δ , using low-energy synchrotron-radiation angle-resolved photoemission. The quantitative relations imply that the distinction between the nodal and antinodal gaps stems from the separation of the condensation and formation of electron pairs, and that the nodal-gap suppression represents the substantial phase incoherence inherent in a strong-coupling superconducting state. These simple gap-based formulae reasonably describe a crucial part of the unconventional mechanism governing T c . In conventional Bardeen–Cooper–Schrieffer (BCS) theory, a superconducting critical temperature T c is proportional to an energy gap, which opens in the electronic excitation spectrum and stands for both the electron-pairing energy and the superconducting order parameter [1] . This proportionality has been considered to break down in high- T c cuprates. As hole concentration p decreases from the optimum, T c decreases, even though the amplitude of d -wave-like gap Δ * increases [2] , [3] . Instead, superfluid density ρ s decreases along with such underdoping, and thus attracted interest as another key parameter for T c [4] , [5] , [6] , [7] , [8] , [9] , [10] . Recently, a variety of experimental gap energies in the superconducting state have been classified into two groups: those that increase like Δ * and those that decrease like T c with underdoping [11] , [12] , [13] . The former energy, Δ * , remains as a pseudogap above T c for the underdoped cuprates, as typically seen in the electronic excitation spectra around an antinode [14] . In the close vicinity of a node, by contrast, the gap closes right above T c , as highlighted by Lee et al . [15] and Pushp et al . [16] The further experimental evidences suggest that the low-energy near-nodal excitations are more relevant to T c than the antinodal ones [16] , [17] . Nevertheless, the gap energies defined under a dichotomy between near-nodal and antinodal regions have been difficult to formulate along with the doping dependences of T c and ρ s [17] , [18] . The unformulated behaviours of the nodal and antinodal gaps posed severe challenges not only to their mutual relationship but also to their standard role in electron pairing. The identities of these gaps have thus been at the center of controversy over a unified picture of the unconventional pairing state in the high- T c cuprates, and intensively examined for clues to the principles underlying the peculiar behaviour of T c . Here we report our finding of simple formulae, based on new experimental data of the nodal gap, Δ N , and the antinodal gap, Δ * , for Bi 2 Sr 2 CaCu 2 O 8+ δ (Bi2212). Clear-cut gap images over the entire Fermi surface have been obtained from low-energy synchrotron-radiation angle-resolved photoemission (ARPES) [19] , [20] , and allowed us to extract the nodal limit of the gap slope beyond the momentum-space dichotomy. As a result, the nodal-gap energy Δ N is reconciled with T c , indicating its relevance to the condensation of the electron pairs. A high plateau value of Δ N / T c ratio exhibits sufficiently strong electron coupling for the underdoped Bi2212. Furthermore, the nodal and antinodal gaps are quantitatively related by a factor of the square-root superfluid density, , in a wide hole-concentration range. This reduction factor is identical to the theoretical prediction for the effect of incoherent pair excitations [21] , [22] , implying that the antinodal gap energy is relevant to the formation of the electron pairs. Thus, we argue that the strong coupling makes a critical difference to the pairing state, and that a substantial number of electrons remain paired, despite dropping out of the coherent superfluid in the underdoped superconducting cuprates. The gap-based formulae shed light on a crucial part of the mechanism governing T c through parameterization with the pairing energy Δ * and the surviving superfluid density ρ s [4] , [5] . 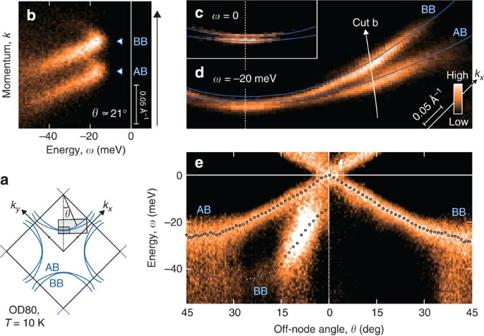Figure 1: Low-energy synchrotron-radiation ARPES data of overdoped Bi2212. The data were collected atT=10 K with a sample ofTc=80 K (OD80) and withhν=8.5 eV. The globally resolved doublet is ascribed to the BB and AB of the CuO2bilayer. (a) Schematic Brillouin zone and off-node angleθabout the (π,π) point. (b) Energy-momentum plot along the off-nodal cut marked by a white arrow in paneld. (c,d) Momentum-space mappings at energies ofω=0 and −20 meV over the fields of view marked by grey rectangles in panela. Blue curves denote the Fermi surfaces determined as minimum-gap loci. (e,f) Energy-verses-θplots of the spectral images along the Fermi surfaces of AB (left) and BB (right), symmetrized with respect toω=0. ARPES data Figure 1 demonstrates that well-defined electronic dispersions were observed throughout the Brillouin zone, and exemplifies extraction of the gap images from a seamless body of ARPES data. The Fermi surfaces were rigorously determined from the minimum-gap loci as marked in Fig. 1b , because both inaccuracy and broadening of the cutting path result in an overestimate of the gap energy. Figure 1c shows that the Fermi surfaces (blue curves) of the bonding band (BB) and antibonding band (AB) of the CuO 2 bilayer are clearly resolved in the momentum space. The spectra were collected along the two Fermi surfaces from the node through to the antinode, and displayed in Fig. 1e as image plots of energy versus off-node angle θ ( Fig. 1a ). The distinct energy splitting seen in Fig. 1e indicates that the BB and AB gaps are resolved in our experiment. Figure 1: Low-energy synchrotron-radiation ARPES data of overdoped Bi2212. The data were collected at T =10 K with a sample of T c =80 K (OD80) and with hν =8.5 eV. The globally resolved doublet is ascribed to the BB and AB of the CuO 2 bilayer. ( a ) Schematic Brillouin zone and off-node angle θ about the ( π , π ) point. ( b ) Energy-momentum plot along the off-nodal cut marked by a white arrow in panel d . ( c , d ) Momentum-space mappings at energies of ω =0 and −20 meV over the fields of view marked by grey rectangles in panel a . Blue curves denote the Fermi surfaces determined as minimum-gap loci. ( e , f ) Energy-verses- θ plots of the spectral images along the Fermi surfaces of AB (left) and BB (right), symmetrized with respect to ω =0. Full size image The comprehensive high-resolution gap study has been supported by low-energy synchrotron radiation [19] , [20] . First, the use of low-energy photons in ARPES experiments facilitates improvement in energy and momentum resolution in compensation for the narrowing of the momentum field of view [15] , [18] , [19] , [20] , [23] . Second, the tunability of synchrotron radiation allows us to optimize the excitation-photon energy hν [19] , [20] . We found that the observability in the off-nodal region is dramatically improved by slightly increasing hν from those used in laser-based ARPES studies, hν ≤7 eV [15] , [18] , [23] . As shown in Fig. 2 , using hν =8.5 eV, the spectral intensities of the BB and AB are sufficient even far off the node, θ ≳ 25°, whereas using hν =7.0 eV, the spectral intensity concentrates only around the node of the AB. Beside the observability, Fig. 2d shows that the spectral peaks for hν =8.5 and 7.0 eV are equally sharp, and that the difference between the BB and AB gaps is insignificant. In the present study, we performed the extensive doping-dependent gap measurements with both hν =8.5 and 7.0 eV, and ruled out unexpected effects of transition matrix elements. 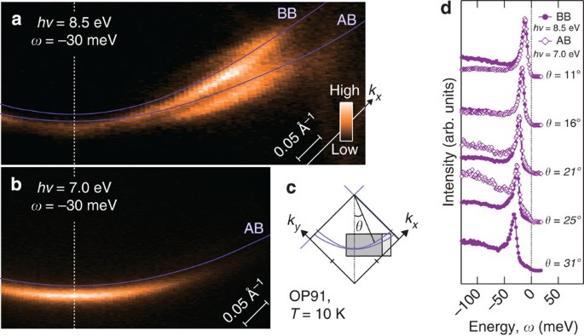Figure 2: APRES data taken with different low-energy photons. The data were collected atT=10 K for an optimally doped Bi2212 withTc=91 K (OP91). (a,b) Momentum-space mappings at an energy ofω=−30 meV, taken withhν=8.5 and 7.0 eV, respectively, over the fields of view marked by grey rectangles inc. Purple curves denote the Fermi surfaces. (c) Schematic of a Brillouin-zone quadrant. (d) EDCs at the minimum-gap loci of the BB (filled circles) and AB (open diamonds), taken withhν=8.5 and 7.0 eV, respectively. Figure 2: APRES data taken with different low-energy photons. The data were collected at T =10 K for an optimally doped Bi2212 with T c =91 K (OP91). ( a , b ) Momentum-space mappings at an energy of ω =−30 meV, taken with hν =8.5 and 7.0 eV, respectively, over the fields of view marked by grey rectangles in c . Purple curves denote the Fermi surfaces. ( c ) Schematic of a Brillouin-zone quadrant. ( d ) EDCs at the minimum-gap loci of the BB (filled circles) and AB (open diamonds), taken with hν =8.5 and 7.0 eV, respectively. Full size image Anisotropic gap evolution Deviation from the d -wave gap is directly imaged in the energy-versus-sin2 θ plots of the ARPES spectra. 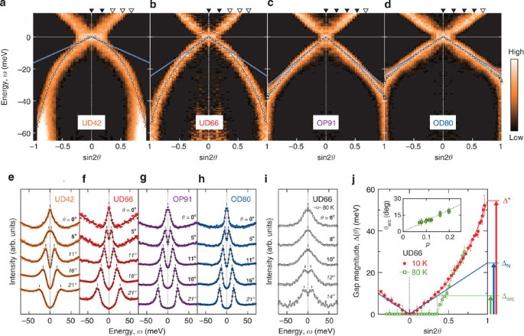Figure 3: ARPES spectra along the Fermi surface for representative dopings. Samples are labelled by a doping-level prefix, namely underdoped (UD), optimum (OP) or overdoped (OD), and a trailing number denotingTc. (a–d) Energy-versus-sin2θplots of the spectral images for BB, taken in the superconducting state atT=10 K and symmetrized with respect toω=0 andθ=0. Circles, curves and blue lines denote the gap energies, the next-higher-harmonic fits and the nodal tangents, respectively. (e–h) EDCs at the momenta marked by triangles in panelsa–d. Black curves and vertical bars denote the fits and the gap energies, respectively. (i) EDCs in the normal state atT=80 K for UD66 (seeSupplementary Fig. S2for other dopings). (j) Gap energies as functions of sin2θin the superconducting (red) and normal (green) states of UD66, determining the energies of antinodal gap Δ*, nodal gap ΔNand arc-endpoint gap Δarc(seeSupplementary Fig. S2for other dopings). Error bars indicate the uncertainty of EDC fit. The inset shows the doping dependence of the Fermi-arc endpoint,θarc, atTTc+10 K alongsideθarc/p=100°(dotted line). The error bars ofθarcstem from the natural broadness of the EDC peaks. The angles inside and outsideθarcare labelled by bold and italic faces ine–i, and marked by filled and open triangles ina–d, respectively. Figure 3a–d reveals that, as hole concentration p decreases from the optimum, the linearity in sin 2 θ becomes severely distorted, making clear a departure from the standard d -wave form, Δ( θ ) sin2 θ , for the underdoped superconducting Bi2212. For in-depth analysis, the gap energies Δ( θ ) were determined by fitting energy-distribution curves (EDCs), and overlaid as small circles in Fig. 3a–d (see Methods). The high fitting quality is presented in Fig. 3e–h , along with typical EDCs (also see Supplementary Fig. S1 ). Here the artifact of the antinodal peak smearing is ruled out of the causes for this deviation [24] , because the curvature in sin 2 θ is established within the region, |sin 2 θ | 0.75, where the well-defined sharp and intense peak is observed for an underdoped sample with T c =66 K (UD66), as shown in Fig. 3b . Figure 3: ARPES spectra along the Fermi surface for representative dopings. Samples are labelled by a doping-level prefix, namely underdoped (UD), optimum (OP) or overdoped (OD), and a trailing number denoting T c . ( a – d ) Energy-versus-sin2 θ plots of the spectral images for BB, taken in the superconducting state at T =10 K and symmetrized with respect to ω =0 and θ =0. Circles, curves and blue lines denote the gap energies, the next-higher-harmonic fits and the nodal tangents, respectively. ( e – h ) EDCs at the momenta marked by triangles in panels a – d . Black curves and vertical bars denote the fits and the gap energies, respectively. ( i ) EDCs in the normal state at T =80 K for UD66 (see Supplementary Fig. S2 for other dopings). ( j ) Gap energies as functions of sin2 θ in the superconducting (red) and normal (green) states of UD66, determining the energies of antinodal gap Δ * , nodal gap Δ N and arc-endpoint gap Δ arc (see Supplementary Fig. S2 for other dopings). Error bars indicate the uncertainty of EDC fit. The inset shows the doping dependence of the Fermi-arc endpoint, θ arc , at T T c +10 K alongside θ arc / p =100 ° (dotted line). The error bars of θ arc stem from the natural broadness of the EDC peaks. The angles inside and outside θ arc are labelled by bold and italic faces in e – i , and marked by filled and open triangles in a – d , respectively. Full size image A key finding from the raw spectral images in Fig. 3a is that the gap deviation penetrates to the close vicinity of the node. The appreciable curvature provides evidence that the gap slope versus sin2 θ smoothly and asymptotically decreases on approaching the nodal limit, θ →0. So far, it has often been assumed that there is some discontinuity between the nodal and antinodal spectra or a certain region with pure d -wave gap [15] , [17] , [18] , [23] , [25] . However, it is difficult to define them with the all-round seamless images in Fig. 3a–d , because the spectral features, such as peak energy, peak width and their derivatives along Fermi surface, gradually change from the antinode to the node [26] . Probably, the nature beyond the simple dichotomy between the near-nodal and antinodal regions comes to light in Bi2212, whose superconducting gap is much larger than that of La 2− x Sr x CuO 4 [25] . The deviation from standard gap behaviour is also deduced from the temperature below which the gap persists, despite the loss of superconductivity. The gap-closing temperature gradually decreases to T c on approaching the nodal limit, θ →0, in a way similar to the deviation from the d -wave gap [15] , [27] . For parameterization of the anisotropic superconducting gap, two methodologies are recognized. One is based on the presence of the pure d -wave region, and to deduce the near-nodal-gap energy from the d -wave fit within such a bounded region [15] , [17] , [18] , [23] , [25] . However, the near-nodal curvatures seen in Fig. 3a hindered us from applying this method to our data, because it would introduce an averaging effect and an extra uncertainty arising from the ill-defined region boundary for the case of the underdoped Bi2212. On this basis, we aimed at the nodal limit of the gap slope in quest of an intrinsic parameter, and adopted the next-higher-harmonic fit over the unbounded region after Mesot et al . [28] and Kohsaka et al . [29] We defined the nodal and antinodal gap energies as and Δ * =Δ( θ )| θ =45° , respectively, so that Δ N /Δ * =1 is satisfied for the ideal d -wave gap as depicted in Fig. 3j . Hence, the fitting function is expressed as where the first term is solely responsible for the nodal-gap slope, the second term models the gap deviation without adjustable angle parameter and its asymptotic behaviour is consistent with the empirical indistinctness of the pure d -wave region. Consequently, as overlaid in Fig. 3a–d , this function well captures the curved gap profiles, Δ( θ ) (solid curves), and their nodal tangents, Δ N sin2 θ (blue lines), for all the doping levels of Bi2212. The shift in focus provides a new perspective on the nodal gap. Dividing the momentum space largely into two half regions, the gap extending over the near-nodal half is less sensitive to underdoping than that in the antinodal half, as seen from Fig. 3a–d . This general trend is consistent with previous reports [16] , [17] , [18] . Combining this trend with the appreciable curvatures observed in Fig. 3a , it follows that the nodal limit of the gap slope, Δ N , decreases with underdoping from OP91 to UD66, and then to UD42, as indicated by blue tangent lines in Fig. 3a–c . The asymptotic behaviour of the gap deviation suggests that the parameter would be purified by taking the nodal limit θ →0. Relation to critical temperature The superconducting-gap energies at various dopings are scaled by T c , and put together in Fig. 4a , which reveals that the nodal limit of Δ( θ )/ T c remains unchanged with underdoping in contrast to the antinodal limit. 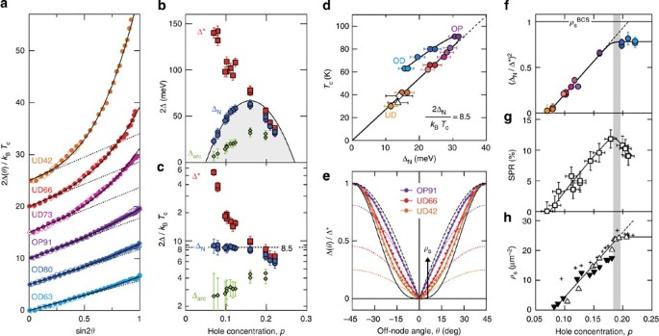Figure 4: Doping dependences of gap parameters. (a) Superconducting-gap energies scaled byTc, plotted as functions of sin2θ, and vertically offset by 5 for each doping. Filled circles denote the BB gap determined withhν=8.5 eV. Open squares and diamonds denote the AB gap determined withhν=8.5 and 7.0 eV, respectively. Solid curves and dotted lines denote the next-higher-harmonic fits and the nodal tangents, respectively. (b) Doping dependences of the energies of nodal gap 2ΔN(blue circles), antinodal gap 2Δ*(red squares), arc-endpoint gap 2Δarc(green diamonds) and 8.5kBTc(black curve). The error bars of ΔNand Δ*derive from the uncertainty of next-higher-harmonic fit. The error bars of Δarcmainly derive from those ofθarc. (c) Same asb, but scaled byTc. (d) Correlation betweenTcand ΔNfor Bi2212 from the present study (coloured circles). Also plotted are the data for optimally doped single-layer cuprates, Bi2Sr2−xLaxCu2Oy(open triangle)23and La2−xSrxCuO4(open diamond)25. (e) Normalized superconducting gaps Δ(θ)/Δ*as functions ofθfor representative dopings. Coloured dotted curves denote the nodal-gap term, ΔNsin2θ. Black dashed and solid curves indicate the gaps expected in the high and low superfluid-density limits, respectively. (f) Square of nodal-to-antinodal gap ratio (ΔN/Δ*)2, which we propose as being proportional toρs21,22. (g) Superconducting-peak ratio (SPR) in the antinodal ARPES spectrum of Bi2212, taken from Fenget al.6. It has been established that SPR is approximately proportional toρs6. (h) Superfluid density,ρs≡λ−2, determined from magnetic penetration depthλwith alternating-current susceptibility (triangles)10and from heat capacity (crosses)7. Figure 4a also shows that the energies of the BB and AB gaps determined with hν =8.5 and 7.0 eV are all consistent with the single fitted-curve for each doping level. The two gap parameters, Δ N and Δ * , determined from the next-higher-harmonic fit are plotted as a function of hole concentration in Fig. 4b . This shows that the nodal gap Δ N closely follows the decrease in T c with underdoping, departing from the antinodal gap Δ * . The gap-to- T c ratios plotted in Fig. 4c are worth noting. As hole concentration p decreases from the overdoped limit, both the nodal and antinodal ones increase with keeping a constant proportion, Δ N =0.87Δ * . This is the canonical behaviour expected when the coupling is getting stronger. A further decrease in p leads to a plateau of 2Δ N / k B T c =8.5, which is about twice the mean-field prediction 4.3 for d -wave weak-coupling superconductors, and meanwhile to a continuing increase in 2Δ * / k B T c [2] , [3] , [13] . These features are beyond the scenario of the standard weak-coupling theory. Figure 4d shows that our data for Bi2212 finely converge on the line of 2Δ N / k B T c =8.5 in particular from the optimum to a heavily underdoped level, and that similar values of 2Δ N / k B T c have been reported for optimally doped single-layer cuprates [23] , [25] . Figure 4: Doping dependences of gap parameters. ( a ) Superconducting-gap energies scaled by T c , plotted as functions of sin2 θ , and vertically offset by 5 for each doping. Filled circles denote the BB gap determined with hν =8.5 eV. Open squares and diamonds denote the AB gap determined with hν =8.5 and 7.0 eV, respectively. Solid curves and dotted lines denote the next-higher-harmonic fits and the nodal tangents, respectively. ( b ) Doping dependences of the energies of nodal gap 2Δ N (blue circles), antinodal gap 2Δ * (red squares), arc-endpoint gap 2Δ arc (green diamonds) and 8.5 k B T c (black curve). The error bars of Δ N and Δ * derive from the uncertainty of next-higher-harmonic fit. The error bars of Δ arc mainly derive from those of θ arc . ( c ) Same as b , but scaled by T c . ( d ) Correlation between T c and Δ N for Bi2212 from the present study (coloured circles). Also plotted are the data for optimally doped single-layer cuprates, Bi 2 Sr 2− x La x Cu 2 O y (open triangle) [23] and La 2− x Sr x CuO 4 (open diamond) [25] . ( e ) Normalized superconducting gaps Δ(θ)/Δ * as functions of θ for representative dopings. Coloured dotted curves denote the nodal-gap term, Δ N sin2 θ . Black dashed and solid curves indicate the gaps expected in the high and low superfluid-density limits, respectively. ( f ) Square of nodal-to-antinodal gap ratio (Δ N /Δ * ) 2 , which we propose as being proportional to ρ s [21] , [22] . ( g ) Superconducting-peak ratio (SPR) in the antinodal ARPES spectrum of Bi2212, taken from Feng et al . [6] . It has been established that SPR is approximately proportional to ρ s [6] . ( h ) Superfluid density, ρ s ≡ λ −2 , determined from magnetic penetration depth λ with alternating-current susceptibility (triangles) [10] and from heat capacity (crosses) [7] . Full size image The proportional relation, 2Δ N =8.5 k B T c , reconciles the critical temperature with the nodal slope of the distorted d -wave superconducting gap. It seems reasonable that T c , in effect, depends on Δ N rather than Δ * , because thermal quasiparticle excitations concentrate in the vicinity of the node and hardly occur around the antinode in particular for the strong-coupling case, 2Δ * / k B T c 4.3. The association between the nodal excitations and T c has been proposed in various ways [12] , [13] , [15] , [16] , [17] . In particular, the decrease in Δ N with underdoping has been deduced from the low-energy slope of B 2g -Raman spectra [12] and the quasiparticle interference in scanning-tunnelling images [29] . Besides, in possible relation to Δ N , the characteristic energies having a p dependence similar to T c have been detected by Andreev-reflection, B 2g -Raman, break-junction-tunnelling and inelastic-neutron-scattering experiments in the superconducting state [11] . Relation to superfluid density An insight comes from the analogy between the doping p and temperature T dependences. The p -dependent distortion of the superconducting gap is presented with normalization to Δ * in Fig. 4e , whereas the T dependence has been reported by Lee et al . [15] With both increasing p and decreasing T , the superconducting gap approaches the ideal d -wave form. As p decreases conversely, Δ N is suppressed relative to Δ*, and decreases towards zero on approaching the disappearance of the superconductivity ( Fig. 4e ). This is analogous to what is observed with increasing T (ref. 15 ). Noting that the superfluid density ρ s decreases towards zero on approaching the critical temperature, T = T c , irrespective of the pseudogap temperature [4] , [5] , [7] , [10] , one may correlate the nodal-gap suppression, Δ N /Δ * , with the decrease in ρ s . In this way, we found another simple relation, . Figure 4f–h compare the square of nodal-to-antinodal gap ratio, (Δ N /Δ * ) 2 , with the superfluid density, ρ s , deduced from the superconducting-peak ratio in antinodal ARPES spectra [6] , and from alternating-current-susceptibility and heat-capacity data [7] , [10] . All of them increase linearly in p with an onset at p ~0.07, showing a saturation point at p ~0.19 (refs 6 , 7 , 10 ). Such a doping dependence of ρ s is known to be universal for the cuprates, and the critical doping of p ~0.19 is not only evident from the superfluid data but has also been identified in the electrical-resistivity and tunnelling data [7] , [13] , [30] . The intimate relationship between the nodal and antinodal gaps is in accord with the continuity between the nodal and antinodal spectra ( Fig. 3a–d ). The square-root dependence on ρ s is usually characteristic of the order parameter, as expected from Ginzburg–Landau theory [1] . More specifically, a general form of has been theoretically predicted for the superfluid reduction due to the incoherent pair excitations inherent in the strong-coupling superconductors, where the degeneracy between the order parameter Δ sc and the pair-formation energy Δ is split, and the former is manifested in the energy of the near-nodal spectral peak as Δ N , whereas the latter dominates the antinodal peak energy Δ * , as shown by taking into account the lifetime effect [21] , [22] . Here the superfluid density in the weak-coupling Bardeen–Cooper–Schrieffer model, , can be regarded as an approximate constant, because the p -dependences of the Fermi-surface perimeter and the normal-state Fermi velocity are relatively small [31] . Therefore, the strong-coupling scenario well explains our empirical relation, , with μm −2 , and is also consistent with the observations of the high gap-to- T c ratios ( Fig. 4c ) and the strong renormalization of dispersion upon the superconducting transition [31] . Under this scenario for the nodal-gap suppression, the phase fluctuation persisting down to a temperature below T c is responsible for the decrease in superfluid density. However, the intrinsic phase fluctuation arising solely from the strong coupling diminishes at temperatures much lower than T c [21] , [22] . Hence, in conjunction with the strong coupling, some extra source generating the incoherent pair excitations at low temperatures is assumed to be present, on the basis of the phenomenology among Δ N , Δ * and ρ s . The possible candidates for this scattering source are the orders competing with the superconductivity [22] . In particular, it has indeed been observed by scanning-tunnelling experiments that the nanoscale spatial domains of density-wave-like modulation spread over the underdoped Bi2212 (ref. 32 ). Perhaps, the limit of 2Δ N / k B T c ≤8.5 may imply that such competing orders are practically inevitable for the strong-coupling superconductivity. Within the weak-coupling scenario, by contrast, there seem no schemes to relate the nodal and antinodal gap energies, to our knowledge. To reconcile 2Δ N / k B T c =8.5 with the weak-coupling constant 4.3, one needs a p -independent reduction factor of ~0.5. The length of ‘Fermi arc’ in the normal state ( Fig. 3i ) seems irrelevant, because of its approximately linear p dependence, θ arc p (see Supplementary Note 1 and Supplementary Fig. S2 ) [15] , [33] , although its experimental uncertainty obscures the behaviour of arc-endpoint gap, Δ arc ≡Δ N sin θ arc ( Fig. 4c ). Furthermore, once in the superconducting state, one cannot distinguish between the spectra at angles θ inside (bold labels) and outside (italic labels) the Fermi arc, as shown in Fig. 3e–h , nor define the boundary of the momentum region with a coherent peak for Bi2212, as pointed out by Vishik et al . [26] Combining the two relations, we obtain . This can be a gap-based formulation of the long-standing phase-fluctuation paradigm that associate T c with both ρ s and the pair-formation energy, (refs 4 , 5 ). Notably, recent investigations have revealed that the rising exponent of T c as a power of ρ s is generally less than 1, and that specifically is satisfied near ρ s =0 (refs 8 , 9 ). This behaviour is compatible with , as far as the variation of Δ * is negligible. Regardless of interpretation, the present phenomenological formulae put strong constraints on existing theories, and provide simple bases for future approaches to the high- T c superconductivity. Samples High-quality single crystals of Bi2212 were grown by traveling-solvent floating-zone method and subjected to a post-annealing procedure for regulation of doping level. An overdoped sample of T c =80 K (OD80), an optimally doped sample of T c =91 K (OP91) and five underdoped samples of T c =81, 77, 73, 66 and 62 K (UD81, UD77, UD73, UD66 and UD62, respectively) were prepared from the crystal whose nominal composition is Bi 2.1 Sr 1.8 CaCu 2 O 8+ δ . Two heavily underdoped samples of T c =42 and 30 K (UD42 and UD30, respectively) were prepared from the Dy-substituted crystal of Bi 2.2 Sr 1.8 Ca 0.8 Dy 0.2 Cu 2 O 8+ δ . Two heavily overdoped samples of T c =73 and 63 K (OD73 and OD63, respectively) were prepared from the Pb-substituted crystal of Bi 1.54 Pb 0.6 Sr 1.88 CaCu 2 O 8+ δ . Details of sample preparation are described elsewhere [34] . Hole concentrations p have been deduced from the samples’ T c , using a phenomenological relation, , from Presland et al . [35] with K. ARPES measurement ARPES experiments were performed on a helical undulator beamline, BL-9A of the Hiroshima Synchrotron Radiation Center, using a SCIENTA R4000 analyzer. Total instrumental energy resolution was set at 5 meV. Clean surfaces were obtained by cleaving the samples in situ , and all the ARPES spectra were collected under ultrahigh vacuum better than 5 × 10 −11 Torr. Energies were calibrated with reference to the intermittently monitored Fermi edge of polycrystalline gold. Fitting EDCs The superconducting-gap energies have been determined by fitting EDCs. For the spectral function A ( ω ) at a minimum-gap locus, we adopted a widely used phenomenological form introduced by Norman et al . [36] , where the peak position and width are given by the superconducting-gap energy Δ and the single-particle scattering rate Γ, respectively. In accordance with the experimental incoherent spectral weight increasing towards higher energies, we added a background linear in energy, a + bω , to A ( ω ), and then applied the multiplication by the Fermi–Dirac distribution function f T ( ω ) as As the experimental antinodal peaks are more asymmetric than the above model function I ( ω ), we additionally used the integral-type background for practical evaluation of the peak position, and applied convolution with the Gaussian representing instrumental resolution. As a result, the fit over a wide energy range of ω ≥−100 meV has been achieved all along the Fermi surface for all the doping levels. The EDCs and their fits are shown in Supplementary Fig. S1 , and those after symmetrization are presented in Fig. 3e–h . As shown by the small circles in Fig. 3a–d , the result of this procedure consistently tracks the spectral peak at the superconducting-gap energy with precision. How to cite this article: Anzai, H. et al . Relation between the nodal and antinodal gap and critical temperature in superconducting Bi2212. Nat. Commun. 4:1815 doi: 10.1038/ncomms2805 (2013).